Solvent-induced immiscibility of polymer brushes eliminates dissipation channels Polymer brushes lead to small friction and wear and thus hold great potential for industrial applications. However, interdigitation of opposing brushes makes them prone to damage. Here we report molecular dynamics simulations revealing that immiscible brush systems can form slick interfaces, in which interdigitation is eliminated and dissipation strongly reduced. We test our findings with friction force microscopy experiments on hydrophilic and hydrophobic brush systems in both symmetric and asymmetric setups. In the symmetric setup both brushes are chemically alike, while the asymmetric system consists of two different brushes that each prefer their own solvent. The trends observed in the experimentally measured force traces and the friction reduction are similar to the simulations and extend to fully immersed contacts. These results reveal that two immiscible brush systems in mechanical contact slide at a fluid–fluid interface while having load-bearing ability. This makes them ideal candidates for tribological applications. An essential function of lubricants is to keep two solids that are in a relative sliding motion from touching directly. Pure water or other fluids that maintain a low viscosity at high pressures do not prevent this microscopic contact formation. Such low-viscosity fluids are squeezed out of the contact as a result of pressure gradients that arise from microscopic surface roughness. This is one reason why commercial lubricants are usually based on oils whose viscosity increases with pressure [1] . Nonetheless, biological lubrication is water based and is able to maintain low friction at all times. Nature accomplishes this type of lubrication by anchoring long, hydrophilic sugar chains to surfaces [2] . These chains swell in an aqueous solvent to form polymer brushes, which can act as a low-viscosity lubricant, even when local pressures are as high as the osmotic pressure of the solvent [3] . In the past two decades, various attempts have been made to mimic the concept of brush-based bio-lubrication in artificial hydrophobic [4] and hydrophilic [5] polymer brush systems, including artificial joints [6] . Friction between two polymer brushes is commonly attributed to direct or hydrodynamic interactions that arise from the overlap of the brushes on opposite sides of the interface [4] , [7] , [8] , [9] , [10] , [11] . Molecular dynamics (MD) simulations have revealed a direct correlation between friction and interdigitation [7] , [8] , [10] , [11] . Experimentally, this finding has been exploited to adjust the overlap and thus the friction between charged brushes, for example, by using electric fields [9] . A critical disadvantage of brush systems is that polymers whose chain termini and loops penetrate the opposing brush are prone to scission and detachment [12] . Here we demonstrate that the overlap of brushes can be avoided. We achieve this in computer simulations and experimentally by bringing a solvated hydrophilic brush into contact with a solvated hydrophobic brush. In these systems, shear is accommodated at a well-defined, slick interface, similar to the contacts between two immiscible, simple liquids [13] . In addition, our contacts can support high normal loads while eliminating the dissipation due to brush overlap. Miscible and immiscible polymer brush systems The principle of our default setups is sketched in Fig. 1 , which shows a symmetric contact with two similar brush systems ( Fig. 1a ) and an asymmetric contact with two immiscible brush systems ( Fig. 1b ). In the experiments, the immiscible brushes are formed by poly(methyl methacrylate) (PMMA) immersed in acetophenone and poly( N -isopropylacrylamide) (PNIPAM) immersed in water. The solvents were chosen for their weak tendency to mix (solubility of 0.55% at 25 o C) and more importantly for their relatively low evaporation rates. PMMA and PNIPAM were grafted from a silicon substrate, and PMMA was grafted from a colloid attached to an atomic force microscopy (AFM) cantilever, with an estimated degree of polymerization of P =7,900 and P =4,000 for PMMA and PNIPAM, respectively. Our simulations [14] are based on the generic Kremer–Grest model [15] , which successfully reproduces the tribological behaviour of adsorbed [16] and end-tethered [8] hydrocarbon films. Our simulation cell contains 250,000 solvent particles and a tip and substrate, each of which carries 4,000 polymers with P =30. In the experiments and simulations shown in Fig. 1 , the brushes were not completely immersed in solvents, to account for the effects of potential contact lines and capillaries. Details on the setups can be found in the Methods section. In the Supplementary Note 1 we show that important dimensionless numbers characterizing the system are of similar order of magnitude, although absolute numbers may differ substantially. For example, the experimental brushes have much larger relaxation times but they are also sheared at distinctly smaller rates than the in silico brushes. Likewise, the ratios of compressed and uncompressed brushes are similar. Given that the simulations hit the correct order of magnitude for the dimensionless numbers, we expect to reproduce the correct trends with our simulations, so that they can be used for the interpretation of experimental results. 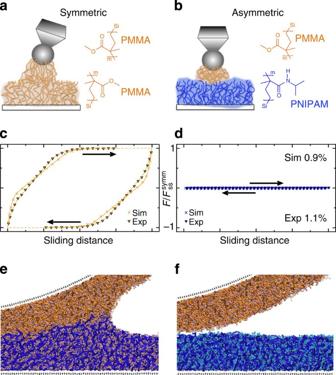Figure 1: Comparison between miscible and immiscible polymer brush systems. The top panels show the schematic setup and chemical formulas of the experimental systems for symmetric (a) and asymmetric (b) contacts. Experimental (triangles) and simulated (crosses) friction traces are shown incanddfor the symmetric and the asymmetric cases, respectively. Friction forcesFare normalized by the steady-state frictionFsssymmof the respective symmetric systems. The solid lines are fits to a shape function, which depends only on two non-dimensional numbers. Snapshots35of the simulation cell are shown ineandf. In the latter, polymers belonging to different brushes are coded with different colours (blue) and (orange), even in the symmetric case, to better visualize the brush overlap. Solvent particles are single coloured in the symmetric case, whereas two coloured in the asymmetric system. Figure 1: Comparison between miscible and immiscible polymer brush systems. The top panels show the schematic setup and chemical formulas of the experimental systems for symmetric ( a ) and asymmetric ( b ) contacts. Experimental (triangles) and simulated (crosses) friction traces are shown in c and d for the symmetric and the asymmetric cases, respectively. Friction forces F are normalized by the steady-state friction F ss symm of the respective symmetric systems. The solid lines are fits to a shape function, which depends only on two non-dimensional numbers. Snapshots [35] of the simulation cell are shown in e and f . In the latter, polymers belonging to different brushes are coded with different colours (blue) and (orange), even in the symmetric case, to better visualize the brush overlap. Solvent particles are single coloured in the symmetric case, whereas two coloured in the asymmetric system. Full size image Figure 1c,d (triangles) shows the measured force traces for a symmetric (PMMA/PMMA) and an asymmetric (PMMA/PNIPAM) system obtained with the same cantilever. In both cases, the surface was moved back and forth by 40 μm at a scan rate of 1 Hz and normal load of 30 nN. The data reveal a friction reduction for the asymmetric system by a factor of 90. The precise value of the reduction varies from surface to surface and depends on the amount of solvent as well as on the normal load. However, the ratio in all our experiments lies between 50 and 130. The friction reduction only weakly depends on the experimental settings (normal load F n , shear rate). For example, for the experimental force traces presented in Fig. 1c,d (colloid diameter 5.8 μm, k n =0.33 N m −1 , k l =61 N m −1 ), we measured for the symmetric system ( Fig. 1c ) a steady-state friction force F ss symm of 170 nN. For the asymmetric system ( Fig. 1d ) we used the same cantilever and experimental settings and we measured a steady-state friction force F ss asymm of 1.85 nN. The friction reduction for this particular experiment was a factor 92. Increasing the shear rate to 5 Hz results in a friction reduction of 90. Increasing the normal load to 300 nN results in a friction reduction of 89. Despite the simplicity of our model, the MD simulations reproduce the experimentally observed trends, as shown in Fig. 1c,d (crosses). First, we again see a reduction in the friction force of roughly two orders of magnitude. Second, the transient responses in the symmetric systems exhibit identical characteristics. There is an initial exponential relaxation of the stress, which is followed by a linear regime that ultimately crosses over to the new steady state through a second exponential relaxation. Third, as shown in Supplementary Fig. 1 , both systems exhibit a similar dip in surface separation shortly after velocity reversal. A differently shaped dip was found in recent MD simulations by Spirin et al. [17] Those simulations were also based on the Kremer–Grest model but performed in a parallel-plate geometry [17] compared with our curved surface geometry. Thus, the shape of the dip appears to be predominantly determined by the geometry of the contact. In the experiments, we observe a small overshoot after the dip that does not occur in the simulations. However, the simulations are based on simple potentials. Moreover, we used chains below the entanglement length. These are two possible explanations for why the overshoot is missing in the simulations. Last, the transient in the asymmetric system is short and can be described by a single exponential in both theory and simulation (see Supplementary Fig. 2 ). Exact quantitative agreement between simulations and experiments cannot be expected because many parameters, such as the respective degrees of polymerization, sliding velocities and pressures, deviate in absolute numbers. Nevertheless, as we tried to keep several dimensionless numbers constant (see Supplementary Note 1 ), we observed the same universal behaviour for each system, that is, the transient response in our symmetric system can be described by the same shape function, which only depends on two dimensionless numbers (see Supplementary Methods ). This agreement is not trivial, as one can see from the qualitative differences not only in the surface dip but also in other response functions that arise solely due to a change in asperity geometry [17] . Given the substantial similarity between the experimental and simulation results, it is justified to further exploit the MD model. The use of the MD model allows us to directly unravel the microscopic details underlying the observed trends in the collective behaviour. In addition, we can extend the simulations to a broader range of parameters and boundary conditions that may be important for practical applications but are difficult to study with the AFM or surface forces apparatus, in particular, the analysis of a velocity range spanning several decades and the analysis of asperity collision. Figure 1e,f reveals that interdigitation is suppressed in the asymmetric system. A sharp interface is formed, across which the solvent velocity u drops discontinuously from 0.8 to 0.2 u (not shown explicitly). This is comparable to the motion of a non-wetting fluid [18] or even a thin gaseous layer [19] past a solid wall. As a consequence, only small shear forces can be exerted across the interface. In contrast, no stratification is observed at the interface of the symmetric system. In the symmetric system, the opposing brushes strongly overlap, and the solvent velocity evolves smoothly across the interface. When the velocity is inverted, the three stages of the transient response correlate with the inversion of the fluid velocity (initial relaxation), the orientation of the polymers (linear regime) and the global shape, so that the entrance of the contact becomes the exit and vice versa (see Supplementary Fig. 3 ). Alternative geometries Thus far, we have considered the motion of a curved solid over a flat substrate. This geometry does not allow us to disentangle the dissipation due to brush overlap and viscoelasticity or to study the effect of capillary formation and break up. However, recent simulations [20] have revealed that these processes are likely to dominate friction at small sliding velocities. To address the question of whether a sharp interface between two immiscible brush systems also reduces dissipation in more general circumstances, we set up a geometry for studying asperity collision. This geometry consists of two periodically repeated cylinders moving either parallel to the symmetry axis ( x direction) or in the transverse y direction (see Supplementary Fig. 4 ). The capillary and viscoelastic dynamics are suppressed for steady-state motion in x . In these simulations, which mimic motion in conformal geometries, friction reduction ( Fig. 2 ) is similar in magnitude but noticeably larger than that in the sphere-plane geometry. The reduction is ≈250 × at the lowest investigated velocities v (10 −4 in Lennard–Jones units, which roughly translates to 1 mm s −1 in real units). Moreover, the friction reduction continues to increase with decreasing velocity because the asymmetric contact exhibits less shear thinning than the symmetric contact. Specifically, the friction coefficient μ of the symmetric contact scales with μ ~ v 0.57 , which is well established for plane-plate geometry sliding [8] , [11] , whereas the asymmetric system obeys μ ~ v 0.88 . Shear thinning in the asymmetric system correlates with a smoothing of the interface and a broadening of the gap. 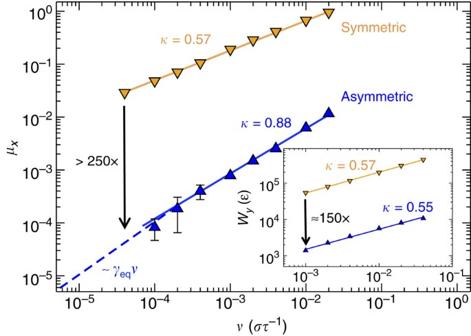Figure 2: Friction coefficients for alternative geometries. The main panel shows the friction coefficientμxversus velocityvfor the symmetric (μx,s, orange symbols) and the asymmetric system (μx,a, blue symbols) on sliding the two cylinders at constant distance (xdirection). The solid lines are power-law fits, resulting in exponents ofκ=0.57 andκ=0.88 for the symmetric and asymmetric contacts, respectively. The dashed line denotes the linear response regime, as extracted from equilibrium runs. At the lowest velocities,μx,ais over 250 × smaller thanμx,s. The inset shows the work per collisionWyversus the velocityvusing the same colour coding as the main graph (orange symbols, data taken from ref.20). For these asperity collisions, we find a friction reduction of 150. Figure 2: Friction coefficients for alternative geometries. The main panel shows the friction coefficient μ x versus velocity v for the symmetric ( μ x ,s , orange symbols) and the asymmetric system ( μ x ,a , blue symbols) on sliding the two cylinders at constant distance ( x direction). The solid lines are power-law fits, resulting in exponents of κ =0.57 and κ =0.88 for the symmetric and asymmetric contacts, respectively. The dashed line denotes the linear response regime, as extracted from equilibrium runs. At the lowest velocities, μ x, a is over 250 × smaller than μ x, s . The inset shows the work per collision W y versus the velocity v using the same colour coding as the main graph (orange symbols, data taken from ref. 20 ). For these asperity collisions, we find a friction reduction of 150. Full size image On sliding in y direction (inset Fig. 2 ), both the symmetric and the asymmetric contact exhibit similar scaling, μ ~ v 0.56±0.01 . Nevertheless, the prefactors differ, and friction is reduced again. The effect even exceeds that for the sphere-on-plane geometry. In fact, our laboratory experiments probed conditions for which the friction reduction is expected to be smallest. The reason is that, for a sphere-on-a-plate geometry, the dominant dissipation channel (viscoelastic brush deformation) cannot be entirely eliminated. Fully solvent-immersed systems It remains to be shown that the method of friction reduction is repeatable, not mainly due to the elimination of the capillary meniscus, and functions for hydrophilic systems too. Towards this goal, additional experiments were conducted in which a PNIPAM brush-bearing colloidal probe, fully immersed in water, was rubbed against a substrate bearing either a fully solvated PNIPAM brush or an acetophenone-saturated PMMA brush. During the exchange, the surfaces were gently dried for a minute with a nitrogen jet and re-solvated with fresh liquid. As revealed in Fig. 3 , the friction reduction is a factor of 50 and thus remains close to two orders of magnitude. Moreover, no signs of performance degradation can be detected even after exchanging the substrate several times. Only after 4 h of sliding, the friction reduction slightly degrades (see Supplementary Fig. 5 ). 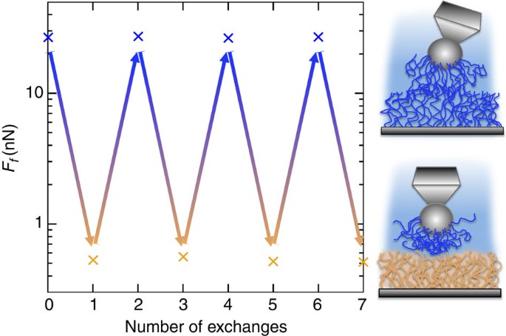Figure 3: Repeatability test for fully solvent-immersed systems. The main panel shows the friction forceFffor the water-immersed symmetric PNIPAM/PNIPAM brush system (top) and the asymmetric PNIPAM/acetophenone-solvated PMMA setup (bottom) on sliding the cantilever at a velocity of 120 μm s−1and a normal load of 180 nN. One data point corresponds to the friction averaged over 512 strokes (1 cycle). After each cycle, the substrate is exchanged by the other solvent-saturated surface and the procedure is repeated. The average friction coefficients are 0.15 and 0.003 for the symmetric and asymmetric systems, respectively. Contact areas and thus normal stresses are difficult to ascertain for our system, but we estimate a lower bound for the pressure of 200 kPa. Figure 3: Repeatability test for fully solvent-immersed systems. The main panel shows the friction force F f for the water-immersed symmetric PNIPAM/PNIPAM brush system (top) and the asymmetric PNIPAM/acetophenone-solvated PMMA setup (bottom) on sliding the cantilever at a velocity of 120 μm s −1 and a normal load of 180 nN. One data point corresponds to the friction averaged over 512 strokes (1 cycle). After each cycle, the substrate is exchanged by the other solvent-saturated surface and the procedure is repeated. The average friction coefficients are 0.15 and 0.003 for the symmetric and asymmetric systems, respectively. Contact areas and thus normal stresses are difficult to ascertain for our system, but we estimate a lower bound for the pressure of 200 kPa. Full size image Finally, we discuss the potential implications of our results for technical applications and a comparison to related systems. The smallest reported friction coefficients for lubricated systems were observed for hydrogels on surfaces at relatively large velocities (1 mm s −1 to 1 m s −1 ) but low pressures (<5 kPa) [21] . A likely reason why friction is smaller in those hydrogel systems than in ours is that their cross-linked networks are stiffer and thus less inclined to viscoelastic hysteresis than our brushes. However, an advantage of our setup is that it functions up to high normal pressures. Zwitterionic brushes also display extremely small friction in aqueous solvents at high normal stresses (7.5 MPa), despite the contacts being symmetric [22] . However, we see signs of damage to the coatings for symmetric systems after long-term sliding, whereas those of the asymmetric contacts appeared to be undamaged under such conditions (see Supplementary Figs 6 and 7 ). Moreover, there are many surfaces that are degraded by water. With our method, neither of the two solvents used needs to be water based. As long as the solvents separate into two phases during contact (even if the solvents mix in the bulk fluid, as additional simulations reveal), there will be no overlap between the polymer brushes. Although it seems intuitive that the interface between repelling components exhibits low friction, many counterexamples exist. For example, an asymmetric contact of dry hydrophilic and hydrophobic brushes results in high friction [23] . In fact, on shearing PMMA on PNIPAM without solvents, we found that the friction was 50% higher compared with dry PMMA on PMMA. Moreover, super-hydrophobic surfaces containing bubble mattresses in water can show greater friction than hydrophilic systems [24] . Furthermore, water confined within a Janus interface can introduce ‘blisters’ resulting in a complex, highly dissipative liquid [25] . Note that a concept similar to ours already exists in nature. After rain, the outer rim of a pitcher plant changes into a slippery surface for insects, with the rim trapping water in its surface grooves [26] . This creates a low-friction surface in combination with the hydrophobic secretion on the feet of the insects [27] . To exploit this mechanism in a controlled fashion, the low-viscosity fluid must remain in contact with the surfaces, even at high pressures, which we achieved by using end-anchored brushes. Materials Chemicals were purchased from Sigma-Aldrich (The Netherlands) and used as received if not stated otherwise. Organic solvents were purchased from Biosolve (Valkenswaard, The Netherlands). Hydrogen peroxide and ethanol were purchased from Merck (The Netherlands). N -isopropylacrylamide (Acros Organics, Belgium) was recrystallized from hexane/toluene. Methyl methacrylate was pressed through on a basic alumina column to remove the inhibitor. Copper bromide (CuBr) was taken up in 98% acetic acid, stirred overnight, filtered, washed with methanol and dried under vacuum. Deionized water from a MilliQ Advantage A 10 purification system (Millipore, Billerica, Ma, USA) was used. Basic aluminium oxide 60 was purchased from Merck KGaA (Darmstadt, Germany). Acetophenone was received from Acros Organics. Preparation of polymer brushes Polymer brushes were grafted from silicon (Si) substrates, from gold-coated substrates (100 nm gold evaporated on Si wafer having a 10-nm chromium (Cr) adhesion layer) and from gold colloidal AFM probes (6 μm diameter, SQube, CP-CONT-Au, NanoAndMore, Spielburg, Germany) by surface-initiated atom-transfer radical polymerization (SI-ATRP). Initiator deposition on silicon surfaces Silicon substrates were first cleaned in piranha solution (7:3 v/v % mixture of H 2 SO 4 (95–98%) and H 2 O 2 (30%)) for a few minutes, rinsed extensively with water, ethanol and dried (piranha solution reacts strongly with organic compounds and should be handled with extreme caution). The dried substrates were placed into a desiccator around a vial containing (3-aminopropyl) triethoxysilane. The desiccator was then evacuated with a rotary vane pump for 15 min and subsequently closed. Vapour deposition was allowed to proceed overnight. In an Erlenmeyer flask, a solution of toluene (40 ml) and triethylamine (40 μl) was prepared and the substrates were immersed into it and 2-bromo-2-methylpropionyl bromide (40 μl) was added dropwise. The reaction was carried out for 4 h, after which the substrates were rinsed with toluene, washed with ethanol and dried under a stream of nitrogen. Initiator deposition on gold surfaces A monolayer solution was prepared with 2-bromo-2-methyl-propionic acid 11-[11-(2-bromo-2-methyl-propionyl-oxy)-undecyldisulphanyl]-undecyl ester in chloroform (20 ml with the concentration of 0.2 mM) [28] . Gold-coated substrates were cleaned first with chloroform, piranha solution and subsequently rinsed with MilliQ water, ethanol and chloroform. The gold colloidal probes were cleaned with ethanol and chloroform, and both substrates were immersed in the initiator solution overnight. Gold-coated flat substrates were used for further characterization. SI-ATRP of PMMA To achieve polymerization, the initiator-covered substrates were placed in dry vials and purged with argon (Ar) for 1 h. The monomer, MMA (10 g, 0.1 mol), was dissolved in the ATRP medium (10 ml methanol/water mixture with ratio 5:1) and the solution was degassed for 2 h. CuBr (145 mg, 1 mmol) and 2,2'-bipyridine (320 mg, 2 mmol) were added to a flask equipped with a magnetic stirring bar, and deoxygenized by three vacuum-Ar backfill cycles. The degassed monomer solution was transferred into the flask and stirred under Ar for another 15 min until a clear brown solution was observed. Afterwards, the polymerization mixture was injected into each reaction vial, adding enough solution to submerge each sample completely. The polymerization was conducted for 40 h at room temperature, after which the samples were removed from the vials and washed with ethanol and chloroform through multiple cycles. Finally, the substrates were dried under a stream of nitrogen. The PMMA brush-modified colloid probes were kept in toluene. SI-ATRP of PNIPAM We followed the procedure described in ref. 29 . The initiator-covered substrates were placed in dry vials and purged with Ar for 1 h. The monomer N -isopropylacrylamide (5.6 g, 50 mmol) and N , N , N′ , N′ , N′′ -pentamethyldiethylenetriamine (320 μl, 0.5 mmol) were dissolved in the ATRP medium (1.6 ml water and 18 ml methanol) and the solution was degassed for 2 h. Concurrently, CuBr (76 mg, 0.5 mmol) was added to a flask equipped with a magnetic stirrer bar and deoxygenized by purging with Ar. The degassed monomer solution was transferred into it and was stirred under Ar for another 15 min until a clear green solution was observed. The polymerization mixture was injected into each reaction vial in a way that each sample was completely submerged. The polymerization was conducted for 1 h at room temperature, and the reaction was terminated by exposing the solutions to air. The samples were subsequently removed from the vials and washed with MilliQ water and an ethylenediaminetetraacetic acid solution to remove all the copper. Fourier-transformed infrared On gold-coated surfaces grazing incidence Fourier-transformed infrared (FTIR) spectra were recorded at room temperature on a Bruker Vertex 70v vacuum FTIR spectrometer equipped with a mercury cadmium telluride detector (angle of incidence 80°, and spectral resolution of 4 cm −1 , 1,024 scans). Background spectra were recorded on a freshly cleaned gold surface. On silicon surfaces, FTIR spectra were recorded using a Biorad FTS-575C spectrometer equipped with a nitrogen-cooled cryogenic mercury telluride detector (spectral resolution of 4 cm −1 , 800 scans). Background spectra were obtained by scanning a freshly cleaned silicon substrate. The spectra can be found in Supplementary Figs 8 and 9 . AFM measurements The AFM experiments are performed on a Multimode V, a vertical-engage scanner and a liquid cell (Bruker, Santa Barbara, CA). The forces are measured with colloidal probes (sQube, NanoAndMore) with an average probe diameter of R =6±0.5 μm. We choose to use non-coated silicon cantilevers, which are less sensitive to environmental changes. This reduced sensitivity allows us to exchange the sample surfaces and switch back and forth between the symmetric and asymmetric system without having to realign the laser or photodetector (and consequently recalibrate the system). The temperature in the AFM head was measured to be constant at 27 °C. During the measurements, we monitor the torsional response of the AFM cantilever under a slightly positive normal force ( F n =2–80 nN), while moving the surface back and forth (triangle wave) at a scan rate of typically 1 Hz in the perpendicular direction with a stroke length of L stroke =20–60 μm. The stroke length is much larger than the swollen brush height of h brush ≈600 nm or the colloidal diameter. We calibrate the normal stiffness of our cantilevers using the thermal noise method as implemented in the Nanoscope 8 software (typically k n =0.4 N m −1 ) and the torsional stiffness and sensitivity using the method of Wagner et al. [30] (typical stiffness k l =65 N m −1 ). After the experiments, the cantilevers are characterized with the high-resolution scanning electron microscope (HR-SEM Zeiss LEO 1550) to obtain the exact dimensions of the colloid and the cantilever (typical length l =470 μm, width w =60 μm and thickness t =3 μm). Given the uncertainties in the dimensions of the probes and the method of calibration, we estimate our uncertainty in the absolute values of the forces to be 30–50%. However, we only compare measurements performed with the same cantilever (at the same shear rate and normal load) such that calibration uncertainties are irrelevant for the determination of the friction reduction. Procedures system under-saturated with solvent Our symmetric system in Fig. 1 consists of a PMMA brush on the colloid and a PMMA brush on the surface. The system is solvated in acetophenone, which is gently applied to the surface with a syringe. After bringing the cantilever in contact with the surface, the acetophenone moves into the brush on the colloid, thereby forming a capillary bridge between the tip and the surface. To create an asymmetric system, we quickly replace the PMMA surface with a PNIPAM brush-covered surface that is solvated in water. We have tested the friction reduction with different combinations of three different cantilevers and three different PMMA and PNIPAM surfaces. We always obtain a friction reduction between 50 and 130 × . Procedures system immersed in solvent Our symmetric system in Fig. 3 consists of a PNIPAM brush on the colloid and PNIPAM brush on the surface. Now, by removing the water, gently drying the surfaces with nitrogen and replacing the PNIPAM surface with a PMMA surface that is solvated in acetophenone, we create the asymmetric system. The system is in both cases completely immersed in water to circumvent the formation of an acetophenone capillary between PNIPAM and PMMA. We observed oscillations in the force traces for the symmetric system of these measurements, which increased in amplitude and wavelength in time and could become asymmetric in the trace and retrace after ~5 min. We always obtain a friction reduction between 40 and 100 × . AFM characterization of the polymer brushes To determine the grafting density ( Γ ) of the polymer brushes, force-distance curves were recorded by AFM on symmetric systems fully immersed in a good solvent. At each arrangement, three curves were analysed and fitted according to de Gennes’ model [31] . PMMA surfaces have a grafting density of Γ =0.24±0.05 chains nm −2 and PNIPAM of Γ =0.31±0.07 chains nm −2 . We determined the brush heights by scratching the surfaces with a needle and obtaining height images of the surfaces by AFM. The measured height for PMMA brush was 236 nm in air and 1,010 nm swollen in acetophenone and for PNIPAM brush 166 nm in air and 532 nm in water at 27 °C. Consequently, we find swelling ratios of 4.2 for PMMA and 3.2 for PNIPAM, in agreement with experimental observations by others at similar grafting densities [32] , [33] . Assuming that the monomer length is ~0.5 nm, we found degrees of polymerization of P =7,900 and P =4,300 for PMMA and PNIPAM, respectively. MD simulations Our simulations are based on the generic bead–spring model (Kremer–Grest) [15] , that is, elastic springs (finitely extensible nonlinear elastic potential), and Lennard–Jones interactions of the functional form V ( r ij )=4 ε ij {( σ ij r ij −1 ) 12 −( σ ij r ij −1 ) 6 }, where r ij is the distance between two interacting (super) atoms. Typical values for the pair-dependent parameters ε ij and σ ij are ε =30 meV and σ =0.5 nm [16] , which we use as units for energy and length. When atoms are supposed to dislike or like each other, forces are set to zero for distances beyond the potential minimum ( r ≥2 1/6 σ ) or r ≥2.5 σ , respectively. One bead represents roughly 3−5 monomers, which motivates our unit choice for the mass of m =10 −22 kg, so that the unit of velocity is v =7 m s −1 . For the simulations, we set up: a sphere on a plate ( Fig. 1 ) or two parallel cylinders with a radius of curvature of R =100 σ (see Supplementary Fig. 4 ) [20] . In the first geometry, we use a flat bottom surface and a cylinder ( R =100 σ ) that is smoothly brought up to zero height at y =0 and y = L ( L is the length of our simulation cell) over 30 σ . This geometry creates an ellipsoidal contact with the long axis in y direction, which reduces circumferential effects and increases our force resolution on sliding in x . Each wall bears 3,828 polymers (degree of polymerization N =30) with a grafting density of α g =0.16 σ −2 , which is ~2.5 × the critical density for brush formation. For each monomer, there is only one solvent atom so that the brush is under-saturated and thus comparable to our experiments and other experiments where the solvent is in equilibrium with the gas phase and condenses into the brush [34] . As a solvent we use dimers, which, compared with monomers, reduces artificial effects due to layering [11] . We choose our Lennard–Jones parameters between the solvent dimers and the (preferred) polymers such that we have good solvent conditions [8] . The simulations are performed in the NVT ensemble. The temperature is kept constant at T =0.6 εk B −1 using a Langevin thermostat that is implemented in the walls and that is applied in the directions perpendicular to the direction of motion such that there is no measurable interference of the thermostat with the (hydro-) dynamics of the system. More details on the specific interaction parameters can be found in ref. 20 . How to cite this article: de Beer, S. et al. Solvent-induced immiscibility of polymer brushes eliminates dissipation channels. Nat. Commun. 5:3781 doi: 10.1038/ncomms4781 (2014).